NHC-Ni(II)-catalyzed cyclopropene-isocyanide [5 + 1] benzannulation Isocyanides are common compounds in fine and bulk chemical syntheses. However, the direct addition of isocyanide to simple unactivated cyclopropene via transition metal catalysis is challenging. Most of the current approaches focus on 1,1-insertion of isocyanide to M-R or nucleophilc insertion. That is often complicated by the competitive homo-oligomerization reactivity occurring at room temperature, such as isocyanide 1,1-insertion by Ni(II). Here we show a (N-heterocyclic carbene)Ni(II) catalyst that enables cyclopropene-isocyanide [5 + 1] benzannulation. As shown in the broad substrate scope and a [ trans- (N-heterocyclic carbene)Ni(isocyanide)Br 2 ] crystal structure, the desired cross-reactivity is cooperatively controlled by the high reactivity of the cyclopropene, the sterically bulky N-heterocyclic carbene, and the strong coordination ability of the isocyanide. This direct addition strategy offers aromatic amine derivatives and complements the Dötz benzannulation and Semmelhack/Wulff 1,4-hydroquinone synthesis. Several sterically bulky, fused, and multi-substituted anilines and unsymmetric functionalized spiro-ring structures are prepared from those easily accessible starting materials expediently. Alkenes and isocyanides are easily accessible primary starting materials that have often been used in both fine and bulk chemical syntheses through insertion, respectively (Fig. 1a-h ) [1] , [2] , [3] , [4] , [5] , [6] , [7] , [8] . Their homo-dimerization and polymerization reactivity often occur readily in the presence of transition-metal salts at r.t. (Fig. 1b, c, e ). Such a high homo-insertion reactivity implies that a selective cross-reaction is difficult to control. The current methods are mostly done indirectly by an in situ generated imidoyl-M species (i.e., a two-steps process) [4] , [8] , either through a 1,1-insertion of isocyanide to the M-R (Type 1: σ-bond insertion, Fig. 1f ), such as L n Ni-R and L n Pd-R from an alkene or by a nucleophilic attack on the electrophilic isocyanide for a subsequent an alkene insertion (Type 2: nucleophilic insertion, Fig. 1g ) [9] , [10] , [11] , [12] , [13] , [14] , [15] , [16] , [17] . There are only handful of examples that can join them together directly. Pioneering examples are those using trienes and cyclobutenes with a stoichiometric amount of Zirconocene and Titanocene complexes [18] , [19] , [20] , [21] , the corresponding catalytic version is still under development. Cyclopropene seems to be an obvious choice for further study, yet isocyanide just served as a ligand in metalloid insertion to cyclopropenes (Fig. 1h ) [22] , and as an additive in Ni(II)/MAO catalyzed ethene polymerization at r.t [23] . Recently, cationic (NHC)Ni(II) has been developed as an efficient and selective catalyst for insertion and cyclopropene rearrangement [24] , [25] , [26] , [27] , [28] . This prompted us to investigate the (NHC)Ni(II) potential in directing a cross-reaction between a cyclopropene 1 and an isocyanide 2 . Fig. 1: Challenges in catalytic intermolecular [5 + 1] benzannulation development by using cyclopropene and isocyanide as a substrate pair. a Transition-metal mediated two-steps alkene-isocyanide insertion strategy. b Pd(II)-catalyzed cyclopropene polymerization, and the dimerization product structure. c Transition-metal catalyzed cyclopropene rearrangement to indene derivatives and subsequent dimerization. d Semmelhack/Wulff 1,4-hydroquinones synthesis. e Ni-catalyzed isocyanide polymerization. f Isocyanide insertion to Ni(II)R bonds for carbonyl derivatives preparation. g Nucleophilic insertion on Ni(II) isocyanide complex. h Isocyanide as a ligand in Pd-catalyzed metalloid insertion to cyclopropenes. i (NHC)Ni(II) catalyzed [5 + 1] benzannulation by cyclopropene and isocyanide. Full size image In this work, instead of developing more practical imidoyl-M generation methods, we explore an alternate strategy that focuses on a formal addition of those two substrates in the absence of an additional component at the end. Here we show a catalytic intermolecular isocyanide-cyclopropene [5 + 1] benzannulation by NHC/NiBr 2 DME/NaBARF (1:1:2) [29] , [30] , [31] , [32] , [33] , [34] , [35] , [36] . This work is the rare C-C forming reaction between electronic neutral cyclopropene and isocyanide (Fig. 1i ). It generally provides ring-expanding rather than the ring-opening products reported in the early 70 s’ that relies on activated cyclopropene [37] . In sharp contrast to those highly competitive homo reactivities of 1 or 2 as shown in Fig. 1 [26] , [32] , [38] , [39] , [40] , [41] , [42] , [43] , [44] , a (hetero)fused aromatic amine product 3 is obtained. That serves as an aza-synthetic alternative to the Dötz benzannulation formed by metal carbene and alkyne, the Semmelhack/Wulff 1,4-hydroquinones synthesis mediated by Cr/Mo/W(CO) n (Fig. 1d ), as well as the catalytic [2 + 2 + 2]/[4 + 2] cycloadditions of π-systems [45] , [46] , [47] , [48] , [49] . This finding also complements the vinyl cyclopropanes [5 + 1] reactions reported recently as well as those imidoyl insertions reactivities [50] , [51] , [52] . Unlike several other intramolecular ring-expanding strategies based on 1 for the syntheses of phenols and saturated N-cycles (e.g., cycloisomerizations of 1 bearing 3,3-dicarbonyl [53] and [4 + 3] cycloadditions of 1 bearing N-heteroaromatics [54] , respectively), our intermolecular strategy offers fused anilines and endocyclic dienes. Overall, it signifies an exciting catalytic synthesis of aromatic products with a broad substrate scope from two structurally diverse and readily accessible substrates. Catalyst development and optimization Inspired partly by the Ni-catalyzed alkene cyanation [55] , and the high structural similarities between the Ni(II)isocyanide and the L.A. activated Ni(II)CN (L.A. = Al, B) [56] , [57] , we surmised that a cyclopropene may undergo an isocyanide addition by a cationic (NHC)Ni(II) under appropriate condition. We commenced our investigation by using 1a and 2a as a substrate pair and the L1 /NiBr 2 DME/NaBARF (in 1:1:2 ratio, See Fig. 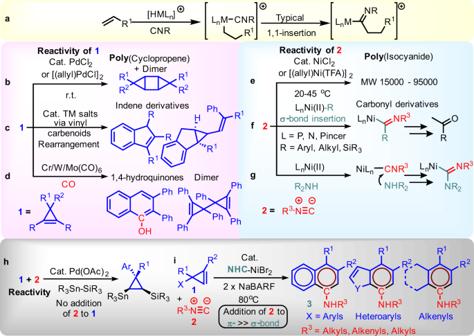Fig. 1: Challenges in catalytic intermolecular [5 + 1] benzannulation development by using cyclopropene and isocyanide as a substrate pair. aTransition-metal mediated two-steps alkene-isocyanide insertion strategy.bPd(II)-catalyzed cyclopropene polymerization, and the dimerization product structure.cTransition-metal catalyzed cyclopropene rearrangement to indene derivatives and subsequent dimerization.dSemmelhack/Wulff 1,4-hydroquinones synthesis.eNi-catalyzed isocyanide polymerization.fIsocyanide insertion to Ni(II)R bonds for carbonyl derivatives preparation.gNucleophilic insertion on Ni(II) isocyanide complex.hIsocyanide as a ligand in Pd-catalyzed metalloid insertion to cyclopropenes.i(NHC)Ni(II) catalyzed [5 + 1] benzannulation by cyclopropene and isocyanide. 2 for L structure) as the catalyst in toluene for 12 hrs at 80 °C (Table 1 , entry 1). Unlike the cross-hydroalkenylation rearrangement reactivity of 1a and alkyne that we anticipated earlier [26] , an aromatic amine 3aa was obtained unexpectedly in ~15% yield rather than other possible acyclic products. The structure of 3aa was confirmed by crystallography, and it highly resembles a 1,4-hydroquinone derived from an LM(CO) n mediated cyclopropene-CO coupling process. Fig. 2: NHC structures employed in this work. NHC L1-7 . DIPP 2,6-diisopropylphenyl. Full size image Table 1 Screening NHC for Ni(II) catalyzed [5 + 1] benzannulation of 1 and 2. Full size table One might envision the [5 + 1] benzannulation of 1 and 2 involved a 6-π electron styrenyl ketenimine rearrangement process [36] (c.f. Figs. 1 d, 3a , typical operation temp: ~120–160 °C bearing electronic activators) [58] , [59] , [60] , [61] instead of an isocyanide addition to an alkene. This is because a relevant styrenyl ketene intermediate can be obtained from 1 by an M(0) oxidative addition [62] , [63] , [64] , [65] and/or acidic metal salts directed rearrangement to the vinylcarbenoid (then Type 3 isocyanide insertion to M(carbene)). So we decided to determine the active components and the catalyst oxidation state that are required for the desired reactivity before optimization. Interestingly, subjecting the independently synthesized styrenyl ketenimines to the (NHC)Ni(0)/(II) at 80 °C conditions did not offer the [5 + 1] benzannulation (Fig. 3b ), and most of the ketenimine was hydrolyzed to amide after 12 hrs. Also, aromatic isocyanides ( 2a , 2b , and 2g , see structure later) did not participate in that reaction in either toluene at 80 °C or refluxing THF for 12 hrs. Indeed, the [5 + 1] benzannulation attempts were unproductive by various (NHC)Ni(0) species, like L1 /Ni(methyl methacrylate) 2 [66] , L1 /Ni(cod) 2 , isolated L1 Ni( 2a ) 3 [67] , and in situ Ni(II) reduction [68] (Table 1 , entry 3). Moreover, common cyclopropene rearrangement products derived from vinylcarbenoid [44] , S E Ar [43] , [69] , σ-bond metathesis or oxidative addition mechanisms, like the 1-methyl indene and indane derivatives 4a′ were not observed as well (Fig. 1c ) [68] , [70] , [71] , [72] , [73] . The major side products obtained from 1 is a mixture of dimer 4a and oligomerization, which contrasts to the M(vinylcarbenoid) mechanism predicted and is similar to the Pd(II) directed dimerization reactivity of 1 at r.t. (Fig. 1b ). In other words, all the above results do not fit the rationale based on a typical 6-π electron styrenyl ketene rearrangement pathway. Thus, the similar performances of the Ni(II)halides were not caused by an unexpected reduction of Ni(II) to Ni(0) (entry 2). And it is not surprising to see a reasonably good reactivity by a L1 Ni(II) at 40 °C, which is supposed to be a less favorable temperature for an oxidative cyclopropene-opening (entry 4 vs Fig. 3 ). Fig. 3: Styrenyl ketene/ketenimine as an intermediate for 6-π electron cyclization. a Dötz Benzannulation and Semmelhack/Wulff synthesis. b 6-π electron cyclization attempts via styrenyl ketenimine. Full size image Control experiments identified that the NHC, the Ni(II) salts, and the NaBArF are all crucial components for the desired reactivity (entry 5-9). In particular, the NaBArF was proved essential for a high catalyst performance (entry 2 vs 5) like the typical Ni(II) catalyzed alkene insertions [74] . Meanwhile, the NHC steric optimization showed an increase in yield and selectivity of 3 (entry 2, 10–15, Fig. 2 , L1 vs L2-3 , L6 vs L7 ). A good balance of desired reactivity and yield was achieved by L7 -NiBr 2 and NaBARF in a 1:2 ratio (entry 16–17), and this catalyst seems promising to cover smaller isocyanides (entry 1 vs 2, 15 vs 18, and 16 vs 19). Such progress was attributed mainly to an optimal steric repulsion among the NHC-Ni(II) and 2 , whereby the strong coordination ability of 2 on cationic (NHC)Ni(II) was fine-tuned, and the desired reactivity of 1 was maintained ( L1-7 ). Thus, a cationic Ni(II) catalyst free of NHC could not provide 3ab from 1a and bulky 2b (entry 9). Ran the reaction in the presence of TEMPO did not result in a significant drop in yield (entry 20, 1:1 to Ni(II)) while using a (IPr)Ni(I)Cl dimer as a catalyst in chlorobenzene only gave <5% desired product (no matter with NaBARF or not, See SI), both results suggesting that Ni(I) was not the active catalyst. By using our optimized catalyst under forcing conditions (i.e., without 2 ), the undesired conversion of 1a was dominated by oligomerization, and dimer 4a was still observed (entry 21) [75] . The [5 + 1] reaction can be done on a larger scale under a slightly modified condition (5 mmol), 1.28 g of 3ab was obtained successfully (81% yield of 3ab , 3 : 4 > 95/5, see SI). Scope of the (NHC)Ni(II) catalyzed [5 + 1] benzannulation With the above basic information in mind, we decided to study the substrate scope and gain mechanistic insight accordingly. First, the scope of 1 was tested by 2b as a substrate pair and L7 /NiBr 2 /NaBArF as a catalyst in toluene at 80 °C for 12 h. To our delight, the scope of R 1 and R 2 on 1 are broad (Fig. 4 ), it offers an exemplary method for making a fused aromatic aniline 3 with various side chains at the p- and m-positions ( 3ab - 3fb ). It covers linear/branch alkyls, functional groups vulnerable to oxidative addition, and radical and nucleophile 2b are compatible (e.g., cyclopropyl and benzyl ether). When a cyclopropene bearing a trisubstituted olefin, the ring-opening event occurs regioselectively, in which only a m- over o-substituted naphthamine regioisomers ( 3eb and 3fb ) was obtained from 1e-f (Trisubstituted olefin with R 1 = H, R 2 = nBu, Aryl = p-C 6 H 4 CF 3 could be used as a pair with 2b at ~120 degree and 20 mol% catalyst loading (see SI, 58% yield, r.r. >95:5)). Besides, ring-strain relief was found as a key factor that governs the reaction [76] , [77] . Terminal alkene near the cyclopropene did not interfere with the desired reactivity and no new cyclopropane was formed there ( 3fb ), suggesting that the postulated Ni(vinylcarbenoid) commonly found in Ni(II) reaction with cyclopropene is not an active intermediate in this reaction again. Fig. 4: Scope of cyclopropene substituents at R 1 and R 2 . Standard condition was followed: IPent An L7 (0.05 mmol), NiBr 2 DME, NaBARF = 1:1:2, cyclopropene 1 : isocyanide 2 = 1:2 (0.5 and 1.0 mmol), at 80 o C in 2 mL toluene for 12 h. Products were characterized by NMR after isolation. Ratio was determined by 1 H NMR. Superscript a indicates 2 mmol of 2 was used. Full size image Such a [5 + 1] reactivity is not limited to 1 bearing an unsubstituted Ph only. Other electronic activated phenyls ( 1g - k ), naphthyl ( 1 l ), and heteroaryls ( 1m - q ) are all possible substrates in this catalysis (Fig. 5a–c ). Electronically activated naphthamines at 5-, 6-, 7-positions, and (hetero)aryl-fused anilines [78] with different relative positions to the NHR were prepared, respectively. This method represents a general route to build several medicinally [79] , [80] , [81] , [82] , [83] , [84] , [85] , [86] , [87] , [88] and photochemically [89] , [90] , [91] important cores bearing different activators and features [92] . Notably, 1r bearing a spiro ring was utilized successfully [93] . That opened up a route to prepare amine-functionalized 2,3-dihydro-1H-phenalenes, a common motif in OLEDs. After a closer look at the results, aromatic substituents on 1 which can donate a higher electron density to the cyclopropene 3-position are more effective substrates. This finding inspired us to consider a cyclopropane ring-strain relief mechanism by the donor-acceptor push-pull reactivity of 1,2-disubstituted cyclopropanes reported in the literature [30] , in which the isocyanide serves as acceptor and the aryl at 3-position serves as a donor (see discussion later). Fig. 5: Scope of cyclopropene substituents at 3-position. Standard condition was followed. Ratio was determined by 1H NMR. a Aryls; b Heteroaryls; c Spiro; d Alkenyl; e Diaryls examples. Superscript a Ratio of 6-:8-OMe regioisomers. b at 60 o C. c 2 mmol of 2 . d 0.5 mmol of 2 was added after 0.5 and 1 h. Full size image The above results in Fig. 4 and Fig. 5a–c implies that the benzannulation scope is not limited to cyclopropene substituted with an aryl. Other electron-donors on the cyclopropene Csp 3 (3-position) that may form the proposed 1,2-disubstituted cyclopropane for the donor-acceptor push-pull reactivity should be a possible substrate of this reaction. 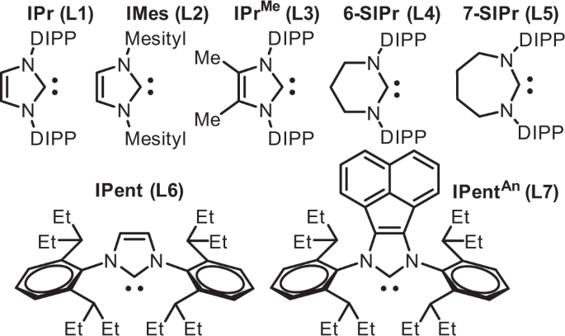Fig. 2: NHC structures employed in this work. NHCL1-7. DIPP 2,6-diisopropylphenyl. Cyclopropenes with simple alkenyls and unsymmetric diaryls at the 3-position were tested next (Fig. 5d, e , 1s - z ), assuming the isocyanide addition selectivity still follows the olefin ring-strain, the vinylcarbenoid formation remains slow, and the isocyanide addition is still accessible even when both the upper and lower sides of 3-position are sterically shielded heavily. Indeed, those substrates followed most of the above assumptions, revealed a route that can prepare alkyl-substituted anilines from non-aromatic cyclopropenes, and 3 substituted with different p-aryl substituents. In particular, cyclic and acyclic alkenyl groups with different substitution patterns are all compatible, 2,4-/3,4-dialkyl substituted anilines from isocyanide directly. Again, no cyclopropanation was detected here, in which a cyclohexenyl group was used to make an aniline fused with cycloalkyl structure ( 3 sb ) and indicated the isocyanide addition selectivity was not simply favored by a cyclic olefin. Up to 95% yield and reasonable π-system selectivity was observed in diaryl examples, despite the steric challenges is high and the electronic differences being moderate. However, the desired product was obtained with a small amount of indene derivative 5 ( 3 : 5 > 95/5). This change in side product preference follows the typical cyclopropene reactivity trend reported in vinylcarbenoid formation literature. Isocyanide scope exploration showed that an optimal steric interaction between the substrate and the NHC is one of the keys for achieving the desired reactivity and selectivity (Fig. 6 ). The L7 can manage isocyanides with distinct and challenging structural characteristics under our standard conditions. The substituent is not limited to simple unfunctionalized phenyl groups, many sterically challenging and electronically diverse groups like unsymmetric and symmetric (hetero)aryls, alkenyls, and alkyls are also compatible. Functional groups sensitive to oxidative and nucleophilic additions in traditional Ni(0)-catalyzed C-N coupling for aromatic amine synthesis, like halides, ester, and nitrile ( 2c-d and 2j-l ), could be used directly without protection. Those groups can serve as versatile handles for reduction and cross-coupling whenever necessary. Undesired reactions like oligomerization of 2 and formation of 5w are more obvious in some less effective pairs. Yet, a higher concentration of 2 improved the yield (e.g., 3wm ), suggesting a high concentration of 2 favors the desired reactivity more than the undesired oligomerization. No amidine and no guanidine product from 2 and 3 was observed in all cases examined, including the sterically less bulky and more electron-rich N-alkyl-N-aryl secondary amines. Thus, both the NH on the N,N-disubstituted amine 3 and the Br are unlikely nucleophilic enough to form an amidinyl and an imidoyl species as the reaction intermediate (c.f. the Type 2 isocyanide insertion). Fig. 6: Scope of aryl, alkenyl, and alkyl-substituted isocyanides. Standard condition was followed. Superscript a 2 mmol of 2 . b Partial hydrolysis of the enamine was observed. 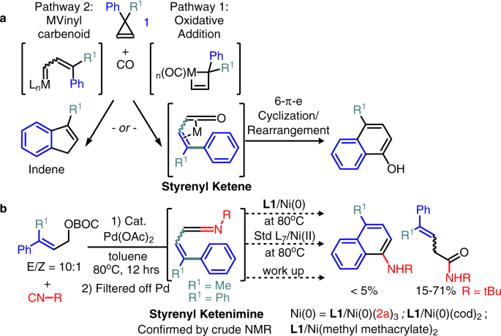Fig. 3: Styrenyl ketene/ketenimine as an intermediate for 6-π electron cyclization. aDötz Benzannulation and Semmelhack/Wulff synthesis.b6-π electron cyclization attempts via styrenyl ketenimine. Yield was determined after complete hydrolysis by stirring in MeOH/H 2 O. Full size image Other than the hints offered by the scope exploration and the relevant literature, several additional experiments were carried out to gain mechanistic insight into the reaction (Fig. 7 ). First, the 5 formation might be caused by the decomposed catalyst at an elevated temperature, since a parallel set of control experiments showed that the 5w was formed mainly by a NiBr 2 DME/NaBARF catalyst free of NHC L7 (Fig. 7a ). This result indicated a strong NHC coordination to a Ni(II) center is important, it could suppress the 3,3-diaryl substituted cyclopropene rearrangement to the corresponding Ni(vinylcarbenoid). Second, we isolated the isocyanide complex (Fig. 7b ). It was prepared in an excess amount of 2b , but the spectroscopic information obtained from the crystal structure revealed a trans-configuration between the NHC and the isocyanide in a 1:1 ratio, and the axial positions are shielded sterically by the isocyanide and the NHC substituents. This complex implied that the NHC can suppress the simultaneous coordination of two isocyanides. Thus, the oligomerization of isocyanide was not observed and manipulations like a slow addition of 2 in a large excess amount are unnecessary for most of our [5 + 1] reactions. Indeed, the typical oligomerization reactivity of 2 , which can be occurred at r.t. by a number of metal salts, is now suppressed appreciably even for 12 h at 80 °C in the presence of NaBArF when an NHC is employed (Fig. 7c ). Next, an IR shift from 2180 to 1940 cm −1 was observed by treating the [ trans -NHC-NiBr 2 ( 2b )] precatalyst with NaBARF (Fig. 7b ). This shift is in agreement with an increase in Ni-CNR backbonding character of a cationic species, rather than the NHC/P-Ni(II)(η 1 -/η 2 -N-aryliminoacyl)Br type of structures at IR range ~1730–1600 cm −1, [94] . The halide abstraction product is quite unstable. Some hydrolysis to amide was indicated by the peaks at ~ 3100, 1850, and 1800 cm −1 region in less than 10 min. No metathesis type of reactivity was observed in the typical [5 + 1] reaction condition. Using two equivalents of NaBArF did not result in a further drop in frequency, and this result supports a mono- rather than di-cationic complex formation [95] . The extra NaBArF employed in the [5 + 1] condition might be used for a better anion exchange efficiency. Interestingly, a 4-phenyl-1-naphthamine derivative, which is similar to our [5 + 1] benzannulation product structure, was obtained successfully from a cyclopropyl carbonitrile alkylation (Fig. 7d ) [76] . This result suggests the donor-acceptor push-pull cyclopropane opening mechanism is plausible for an aryl and CNR substituted cyclopropane as Fig. 5a–c suggested, and the isocyanide addition to the olefin on the cyclopropene is likely involved. Trapping the intermediate from a reaction between 1a and a cationic [(NHC)Ni(allyl)]BArF with D 2 O showed a D-labeled allylcyclopropane with syn-configuration. This result suggests a cyclopropene can undergo insertion like the other alkenes with (NHC)Ni(II), and it may be one of the possible pathways for introducing the (NHC)Ni(II)-CNR (1.844(2) Å from Fig. 7b ) to the cyclopropene. Fig. 7: Mechanistic studies and reaction models. a Effect of NHC and the three-substituent on indene derivative formation; b [ trans -IPr-NiBr 2 (CNDIPP)] crystal structure, IR studies, and NaBArF effect; c NHC effect on 2b oligomerization; d A cyclopropyl carbonitrile alkylation directed rearrangement; e Syn-addition of a cationic (NHC)Ni(II) species to cyclopropene. Full size image At this stage, the keys for the desired [5 + 1] reactivity and broad scope are attributed mainly to the high reactivity of an isocyanide addition to the cyclopropene π-bond by a cationic NHC-Ni(II) catalyst, and the high rearrangement reactivity after that (Fig. 8a ). By the optimal coordination ability and steric effect from NHC, isocyanide and cyclopropene combinations, other typical pathways related to the acidic metal salt directed vinylcarbenoid formation and oligomerization are suppressed accordingly. One of the possible reaction sequences may involve a cationic (NHC)Ni(II) directed addition of 2 to 1 , similar to P-Pd(II)acetylide insertions to alkenes and resemble hydro-/alkyl-nickelation to 1 (Fig. 1 a, 3 ) [32] , [96] , [97] . It may be assisted by (a) an optimal steric repulsion between NHC and 2 (otherwise NHC-Ni(II)(η 2 -iminoacyl) complex can be formed at −35 °C by isocyanide 1,1-insertion), (b) a halide abstraction by NaBArF [14] , [98] , [99] , [100] , and (c) a lowered vinylcarbenoid formation and oligomerization reactivity of 1 in the presence of strongly coordinating 2 and NHC (Table 1 , entry 21) [101] . Next, a ring-strain relief triggered dearomatization may occur (Int.-1) [76] , [77] , similar to the donor-acceptor push-pull reactivity of 1,2-disubstituted cyclopropanes [30] . The substituent repulsions between the bulky L7 and the cyclic tether from 1 may restrict the Int.-2 conformation. Hence, the ketenimine and the cyclic tethers were aligned on the same side, and the competing styrenyl ketenimine formation pathway was suppressed (See SI for details). Since the postulated Int.-2 has no β-H available for the Ni(II), ligand exchange with another 2 may facilitate the ring closure (Int.-3) and regenerate the catalyst. After a facile re-aromatization over imine hydrolysis, those highly substituted 3 can be formed. Fig. 8: Working hypothesis of the cyclopropene and isocyanide [5 + 1] reactions by a (NHC)Ni(II) catalyst. a Benzannulation. b 1,3-Diene substituted spiro-rings. Postulated structures are in brackets, and the anion is omitted for clarity. Full size image Based on the working hypothesis, a catalytic [5 + 1] endocyclic diene synthesis was also achieved (Fig. 8b, 8ab-db ) by intercepting the postulated re-aromatization step (Int.-3 to 3 ). Unsymmetrically substituted spiro-ring structures were obtained from the corresponding 7 and 2 in just a step by the standard condition (e.g., spiro[4,5]deca-dien-imine), in which heterocycles are also tolerated. Notably, by a comparison of the side chains on cyclopropene 1 and 7 , the above examples do not support a [5 + 1] mechanism initiated by an aryl side chain imidoylation (by CH activation, then 1,1-insertion of 2 ). That is simply because the alkenyl side chain on 7 has no H at the β-position. Regioselective post-modifications Finally, the product 3 can serve as a key building block for a higher substituted aromatic amine synthesis easily. For instance, a solvent-controlled highly regioselective bromination on unsymmetric diaryl amine was achieved by simply using NBS as Br source (Fig. 9 , ratio was determined by GCMS) [102] , [103] . These functionalized sites may serve as additional handles for preparing other related structures with similar sets of cores. Fig. 9: Post-modification of the product. Solvent-controlled regioselective bromination on unsymmetrically substituted diaryl amine. Full size image We have developed an intermolecular cyclopropene-isocyanide [5 + 1] benzannulation by a cationic NHC-Ni(II) catalyst with a BArF anion, in which those two substrates were unreactive to each other before and were dominated by their own reactivities. These combinations showed the strength of this catalyst design in broadening the use of those structurally diversified starting materials with remarkably good functional group compatibilities and regulating competitive reactivities of those two substrates at an elevated temperature. This method serves as an aza-synthetic alternative for products structurally similar to those in Dötz benzannulation and Semmelhack/Wulff synthesis based on Cr/Mo/W(CO)n as well as those in styrenyl ketene 6-π electron cyclizations. The study also provides a method to make unsymmetric and functionalized spiro-ring structures catalytically. This work has revealed several opportunities to utilize isocyanide and cyclopropene for other potential applications. 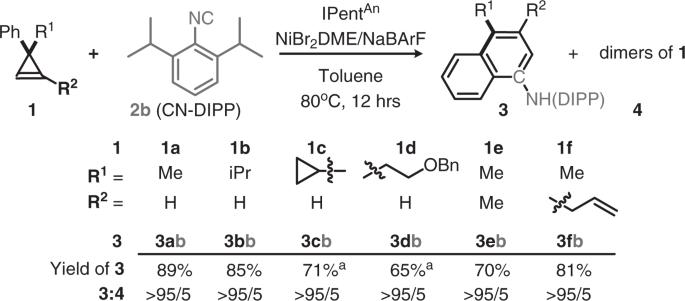Fig. 4: Scope of cyclopropene substituents at R1and R2. Standard condition was followed: IPentAnL7(0.05 mmol), NiBr2DME, NaBARF = 1:1:2, cyclopropene1: isocyanide2= 1:2 (0.5 and 1.0 mmol), at 80oC in 2 mL toluene for 12 h. Products were characterized by NMR after isolation. Ratio was determined by1H NMR. Superscriptaindicates 2 mmol of2was used. General procedure for the [5 + 1] Benzannulation To a catalyst mixture (0.05 mmol L7 /NiBr 2 DME, 0.10 mmol NaBARF) stirred in toluene (1 mL) for 3 min at 80 o C, an indicated amount of a premixed toluene solution of 1 and 2 (1 mL) was added in one-pot and stirred for an additional 12 h. After cooled down to r.t., it was diluted with 6 mL nhex/EA (10:1) and filtered through a short plug of silica gel. The solvent was then removed on rotavap. Conversion of 1 and selectivity of 3 to other possible isomers were determined by 1 H NMR or GCMS (average of two runs). 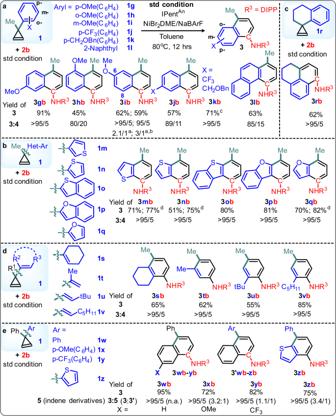Fig. 5: Scope of cyclopropene substituents at 3-position. Standard condition was followed. Ratio was determined by 1H NMR.aAryls;bHeteroaryls;cSpiro;dAlkenyl;eDiaryls examples. SuperscriptaRatio of 6-:8-OMe regioisomers.bat 60oC.c2 mmol of2.d0.5 mmol of2was added after 0.5 and 1 h. 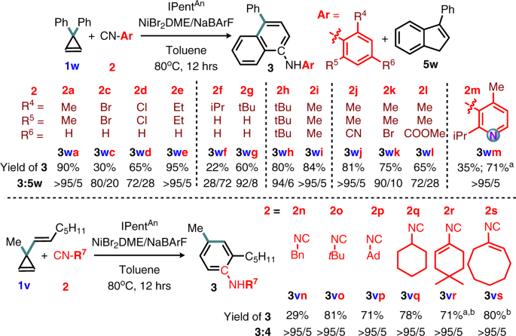Fig. 6: Scope of aryl, alkenyl, and alkyl-substituted isocyanides. Standard condition was followed. Superscripta2 mmol of2.bPartial hydrolysis of the enamine was observed. Yield was determined after complete hydrolysis by stirring in MeOH/H2O. 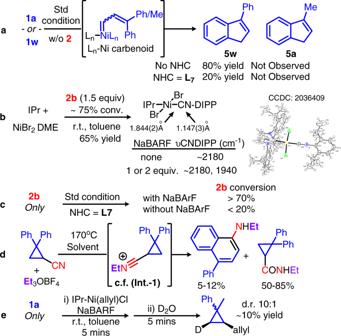Fig. 7: Mechanistic studies and reaction models. aEffect of NHC and the three-substituent on indene derivative formation;b[trans-IPr-NiBr2(CNDIPP)] crystal structure, IR studies, and NaBArF effect;cNHC effect on2boligomerization;dA cyclopropyl carbonitrile alkylation directed rearrangement;eSyn-addition of a cationic (NHC)Ni(II) species to cyclopropene. 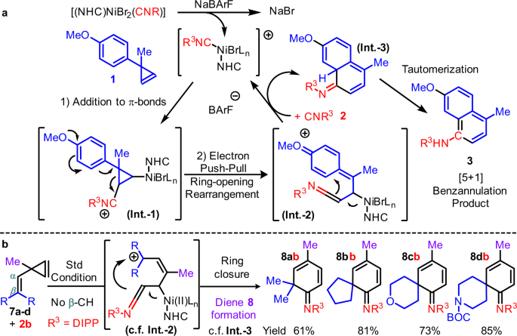Fig. 8: Working hypothesis of the cyclopropene and isocyanide [5 + 1] reactions by a (NHC)Ni(II) catalyst. aBenzannulation.b1,3-Diene substituted spiro-rings. Postulated structures are in brackets, and the anion is omitted for clarity. 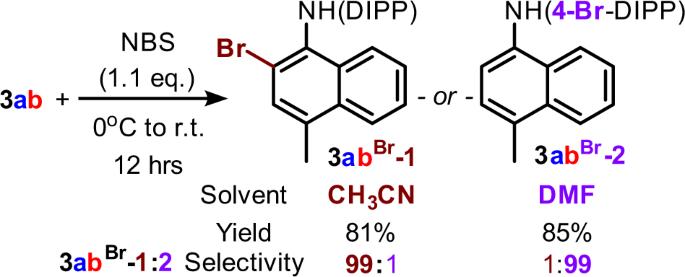Fig. 9: Post-modification of the product. Solvent-controlled regioselective bromination on unsymmetrically substituted diaryl amine. Product structures were confirmed by chromatography and isolation (5–10% EA/Hex).